5-Hydroxymethylcytosine in the mammalian zygote is linked with epigenetic reprogramming The epigenomes of early mammalian embryos are extensively reprogrammed to acquire a totipotent developmental potential. A major initial event in this reprogramming is the active loss/demethylation of 5-methylcytosine (5mC) in the zygote. Here, we report on findings that link this active demethylation to molecular mechanisms. We detect 5-hydroxymethylcytosine (5hmC) as a novel modification in mouse, bovine and rabbit zygotes. On zygotic development 5hmC accumulates in the paternal pronucleus along with a reduction of 5mC. A knockdown of the 5hmC generating dioxygenase Tet3 simultaneously affects the patterns of 5hmC and 5mC in the paternal pronucleus. This finding links the loss of 5mC to its conversion into 5hmC. The maternal pronucleus seems to be largely protected against this mechanism by PGC7/Dppa3/Stella, as in PGC7 knockout zygotes 5mC also becomes accessible to oxidation into 5hmC. In summary, our data suggest an important role of 5hmC and Tet3 for DNA methylation reprogramming processes in the mammalian zygote. Genome-wide reprogramming of DNA methylation (5-methylcytosine; 5mC) is an important epigenomic process observed in mammalian primordial germ cells and early embryos. The reprogramming of DNA methylation has a direct influence on genomic imprints, the regulation of pluripotency and stem cell networks, the erasure of epimutations and the transcriptional control of transposons [1] , [2] , [3] . In the mammalian zygote, the 5mC content of the paternal chromosomes is substantially reduced before replication of DNA, as detected by immunofluorescence (IF) imaging with antibodies against 5mC [4] , [5] , [6] , [7] . Several lines of evidence suggest that the conversion of 5mC to cytosine can be induced by deamination followed by DNA glycosylase-induced base excision repair [8] , [9] , [10] . We recently analysed the dynamics of active loss/demethylation of 5mC using bisulphite sequencing on staged mouse zygotes. We could indeed find a potential link between 5mC demethylation and base excision repair. In addition, we reported that the loss of 5mC is less pronounced compared with the extensive signal reduction observed by IF with antibodies against 5mC [7] . The latter observation prompted us to search for additional mechanisms that may contribute to the zygotic loss of 5mC. The recent detection of 5-hydroxymethylcytosine (5hmC) in Purkinje and embryonic stem (ES) cells, strongly suggests that this modification could indeed have an intermediate function in reprogramming of 5mC [11] , [12] . The extensive conversion of 5mC into 5hmC in the zygote would explain the rapid loss of 5mC IF signal, while at the same stages we see a remarkable maintenance of modifications at cytosines using sodium bisulphite sequencing. Note that both modifications, 5mC and 5hmC, are resistant to bisulphite induced deamination and thus cannot be discriminated in bisulphite sequencing reactions [13] . The presence of 5hmC has not been examined in zygotes. 5hmC can be formed by hydroxylation of 5mC by the dioxygenases Tet1, Tet2 and Tet3. Tet1 expression was reported in the zygote and a knockdown of Tet1 during early embryogenesis revealed effects on inner cell mass specification [14] . In this paper, we describe a detailed analysis of 5hmC distribution in mouse and other mammalian zygotes, as well as in cloned embryos. We also analysed the effect of Tet1-3 ablation and the absence of the protective factor PGC7 on the dynamics of 5hmC and 5mC in the maternal and paternal pronuclei of the developing mouse zygote. Our findings point towards a major role of 5hmC in the process of epigenetic reprogramming during the earliest phase of development and open new perspectives on the mechanisms of active DNA demethylation. Dynamic appearance of 5hmC during zygotic development We first investigated the presence of 5hmC using several polyclonal and monoclonal antibodies raised and tested against 5hmC (see Methods for details). All antibodies show a strong reactivity in advanced mouse zygotes ( Fig. 1a ; Supplementary Fig. S1 ). 5hmC signals are most prominent in the paternal pronucleus, in which the reactivity against 5mC antibody is already weak. The opposite patterns are found in the maternal pronucleus. Here, strong staining by the 5mC antibody is accompanied by a much less intense 5hmC signal. The 5mC content of the paternal pronucleus is known to dynamically change over the first cell cycle. We followed the dynamics of 5hmC in comparison to 5mC patterns across all pronuclear stages of the zygote (see Fig. 1b for an example of 5hmC). The relative changes within the paternal and maternal pronuclei, respectively, were determined by image quantification using standardized fixation, denaturation and imaging conditions ( Fig. 1c–f ). At the earliest developmental stages after sperm entry (PN0 and PN1) both compact pronuclei show 5hmC and 5mC signals of similar intensities. On further development the distribution, intensities and ratios of 5hmC and 5mC signals become increasingly different for maternal and paternal pronuclei, respectively, towards the end of the first cell cycle ( Fig. 1b–f and Supplementary Fig. S2 ). The 5hmC signal steadily increases in the paternal pronucleus by about sevenfold at late PN3 (beginning of S-phase), whereas the 5mC signal decreases. Similar, but much less pronounced changes are detectable in the maternal pronucleus. Here, the 5hmC signal increases moderately (about twofold at PN3), whereas the 5mC signal decreases slightly. This decrease of the maternal 5mC content has not been documented before; it only becomes evident when quantifying the relative 5mC intensities normalized against DNA antibody signals. 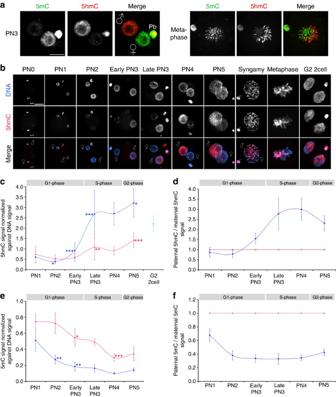Figure 1: 5hmC preferentially appears in the paternal genome of early mouse preimplantation embryos. (a) Representative images of mid PN3 and metaphase stage zygotes stained with 5-methylcytosine (5mC, green mouse monoclonal, gift from Dirk Schübeler) and 5-hydroxymethylcytosine (5hmC, red rabbit polyclonal from Active Motif) antibodies. (b) Dynamic appearance of 5hmC during early preimplantation development. Shown are representative images of embryos stained with DNA (blue mouse monoclonal from Millipore) and 5hmC (red rabbit polyclonal from Active Motif) antibodies. (c) Quantification of 5hmC signal normalized against DNA antibody signal. A total of 12–18 precisely staged embryos per pronuclear stage from 3 to 5in vitrofertilization (IVF) experiments were analysed. (d) Comparison of paternal and maternal 5hmC signal (maternal signal set to 1) normalized against DNA antibody signal. (e) Quantification of 5mC signal normalized against DNA antibody signal. A total of 3–9 precisely staged embryos per pronuclear stage from 2 to 3 IVF experiments were analysed. (f) Comparison of paternal and maternal 5mC signal (maternal signal set to 1) normalized against DNA antibody signal. Asterisks show significant changes of paternal or maternal 5hmC/5mC signals calculated using Student'st-tests (*=P<0.05, **=<0.01, ***=P<0.001). Error bars represent standard deviations. Blue line, paternal; red line, maternal signal; ♂, male; ♀, female pronucleus; Pb, polar body; scale bar, 20 μm. Figure 1: 5hmC preferentially appears in the paternal genome of early mouse preimplantation embryos. ( a ) Representative images of mid PN3 and metaphase stage zygotes stained with 5-methylcytosine (5mC, green mouse monoclonal, gift from Dirk Schübeler) and 5-hydroxymethylcytosine (5hmC, red rabbit polyclonal from Active Motif) antibodies. ( b ) Dynamic appearance of 5hmC during early preimplantation development. Shown are representative images of embryos stained with DNA (blue mouse monoclonal from Millipore) and 5hmC (red rabbit polyclonal from Active Motif) antibodies. ( c ) Quantification of 5hmC signal normalized against DNA antibody signal. A total of 12–18 precisely staged embryos per pronuclear stage from 3 to 5 in vitro fertilization (IVF) experiments were analysed. ( d ) Comparison of paternal and maternal 5hmC signal (maternal signal set to 1) normalized against DNA antibody signal. ( e ) Quantification of 5mC signal normalized against DNA antibody signal. A total of 3–9 precisely staged embryos per pronuclear stage from 2 to 3 IVF experiments were analysed. ( f ) Comparison of paternal and maternal 5mC signal (maternal signal set to 1) normalized against DNA antibody signal. Asterisks show significant changes of paternal or maternal 5hmC/5mC signals calculated using Student's t -tests (*= P <0.05, **=<0.01, ***= P <0.001). Error bars represent standard deviations. Blue line, paternal; red line, maternal signal; ♂, male; ♀, female pronucleus; Pb, polar body; scale bar, 20 μm. Full size image Both pronuclei not only differ in the signal intensities, but also the distribution of 5hmC signals up to late S-phase. Although 5hmC stains the paternal genome across the entire pronucleus, the signal in the maternal one is concentrated in heterochromatic rings around nucleolar precursor bodies. During S-phase the paternal 5hmC content remains about threefold higher than the maternal one ( Fig. 1d ). In G2-phase (PN5), the 5hmC signals reach their maximum in both pronuclei ( Fig. 1c ). At metaphase, the arms of the paternal chromosomes are strongly stained for 5hmC in contrast to maternal chromosomes, on which the 5mC signal predominates. An exception is the pericentromeric regions, which on both maternal and paternal chromosomes retain a strong 5mC signal ( Fig. 1a ). This indicates that parental chromosomes not only differ in the quantity, but also in the relative distribution of 5mC and 5hmC. The parental differences in 5hmC apparently persist into the 2-cell stage. Here, nuclear regions with a stronger 5hmC stain most likely demarcate the territory of still separated paternal chromatin (see Fig. 1b ). The image processing of nuclei of late 2-cell embryos (in G2-phase), which have completed the second round of replication, reveal that 2-cell embryos retain approximately the same 5hmC signal intensities as PN5 pronuclei (G2-phase) of the zygote. Thus, unlike in the first cell cycle, the 5hmC content is not further altered (neither increased nor decreased) during G1 and S-phase of 2-cell embryos. In line with this, we observe a strong decrease of Tet3 expression in 2-cell embryos (see below). Accumulation of 5hmC is independent of DNA replication In the paternal pronucleus, 5hmC begins to accumulate at early to mid PN3, that is, before replication commences. The strongest increase, however, is detectable during S- and G2-phase. This led us to investigate, whether the appearance of 5hmC is dependent on DNA replication. Zygotes incubated with aphidicolin from late G1-phase onwards do not replicate their DNA (no EdU or BrdU incorporation, see also Wossidlo et al ., [7] Fig. 3). However, the drug does not inhibit DNA decondensation and pronuclear progression to PN5 morphology ( Supplementary Fig. S3 ). In aphidicolin-treated late stage zygotes, 5hmC intensities and their pronuclear distribution are not changed compared with control mock-treated zygotes ( Supplementary Fig. S3 ). We conclude that the accumulation of 5hmC occurs independently of DNA replication. Antibody independent analysis of the presence of 5hmC in zygotes To obtain independent experimental proof for the presence and dynamics of 5hmC in zygotes, we developed a nuclease-based in situ assay using the nuclease McrBC. McrBC was originally described to preferentially cut 5hmC containing DNA in comparison to 5mC [15] (see also Supplementary Fig. S4a ). Following McrBC in situ digestion the DNA ends are marked by TUNEL (terminal deoxynucleotidyl transferase dUTP nick-end labelling, modified HELMET assay [16] , see Supplementary Methods ). McrBC TUNEL label increased in developing paternal pronuclei compared with maternal ones, whereas TUNEL signals were equal for both at early PN2 stages (see Supplementary Fig. S4b,d for quantification). Hence, the relative changes and dynamics in 5hmC observed by IF could be recapitulated by an independent assay (see also Supplementary Fig. S1 ). 5hmC is present in rabbit and bovine zygotes Following our observations in mouse, we also examined the presence of 5hmC in rabbit and bovine zygotes, that is, two other mammals reported to show paternal DNA demethylation (see Supplementary Fig. S5 and refs. 5 , 17 ). In both bovine and rabbit zygotes, we find a similar inverse 5mC and 5hmC staining in the paternal and maternal pronuclei, respectively ( Fig. 2 and Supplementary Fig. S5 ). We conclude that the asymmetric 5hmC presence is conserved in three mammalian species pointing towards a conserved role of 5hmC in epigenetic reprogramming. 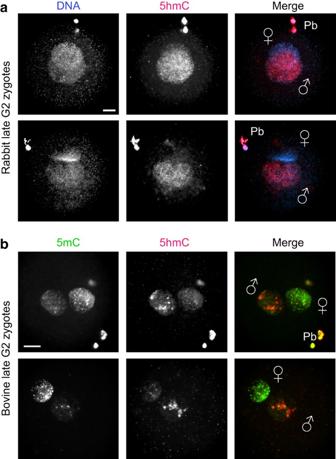Figure 2: 5hmC is present in rabbit and bovine zygotes. Representative images of (a) rabbit and (b) bovine G2-phase zygotes stained with 5hmC (red rabbit polyclonal from Active Motif) and DNA (blue mouse monoclonal from Millipore)/5mC (green mouse monoclonal, gift from Dirk Schübeler) antibodies (N>10). ♂♂,male pronucleus; ♀, female pronucleus; Pb, polar body; scale bar, 20 μm. Figure 2: 5hmC is present in rabbit and bovine zygotes. Representative images of ( a ) rabbit and ( b ) bovine G2-phase zygotes stained with 5hmC (red rabbit polyclonal from Active Motif) and DNA (blue mouse monoclonal from Millipore)/5mC (green mouse monoclonal, gift from Dirk Schübeler) antibodies ( N >10). ♂♂,male pronucleus; ♀, female pronucleus; Pb, polar body; scale bar, 20 μm. Full size image 5hmC in embryos derived by somatic cell nuclear transfer We next examined the dynamics of 5hmC in chromosomes of one-cell embryos obtained after somatic cell nuclear transfer (SCNT). Cloned one-cell embryos (with cumulus cells as donors) were stained for 5mC and 5hmC at 2, 6 and 12 h post-activation (hpa; Fig. 3 ). At 2 hpa strong distinct foci of both 5mC and 5hmC are present in the two pseudo-pronuclei formed after cumulus cell nuclear transfer. Note that the remaining two spindles in the enucleated oocyte lead to the formation of these two pseudo-pronuclei. Also note that cumulus cells apparently contain a substantial amount of 5hmC. As in zygotes, the 5hmC signal decreases during the first few hours of development of the cloned embryos (up to 6 hpa, late G1-phase) and is followed by an S-phase associated increase reaching high levels at 12 hpa (that is, at early G2-phase). Conversely, the 5mC signal decreases during development of SCNT embryos ( Fig. 3 and see refs. 5 , 7 ). The accumulation of 5hmC in nuclei of SCNT one-cell embryos not only confirms the modification processes that occur in zygotes derived by in vitro fertilization (IVF), but also suggests that an enzymatic activity required for the formation of 5hmC is provided by the oocyte cytoplasm. 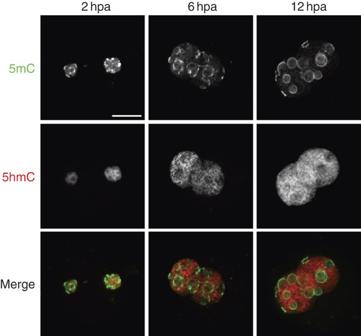Figure 3: 5hmC in somatic cell nuclear transfer (SCNT) derived one-cell embryos. Representative images of 2, 6 and 12 h post-activation (hpa; early G1-, late G1- and early G2-phase, see ref.7) SCNT derived one-cell embryos stained with 5mC (green mouse monoclonal, gift from Dirk Schübeler) and 5hmC (red rabbit monoclonal from Active Motif) antibodies (N>35). Scale bar, 20 μm. Figure 3: 5hmC in somatic cell nuclear transfer (SCNT) derived one-cell embryos. Representative images of 2, 6 and 12 h post-activation (hpa; early G1-, late G1- and early G2-phase, see ref. 7 ) SCNT derived one-cell embryos stained with 5mC (green mouse monoclonal, gift from Dirk Schübeler) and 5hmC (red rabbit monoclonal from Active Motif) antibodies ( N >35). Scale bar, 20 μm. Full size image Expression levels of Tet proteins in oocytes and embryos The most parsimonious explanation for the generation of 5hmC in the zygote is that it is produced by the hydroxylation of 5mC by the Tet enzymes [12] , [14] . 5hmC, however, can in theory also be generated independently of 5mC [18] . We investigated the potential involvement of the Tet enzymes in this process. Quantitative reverse transcription PCR (qRT–PCR) revealed that transcripts for Tet1, 2 and 3 are differentially expressed in oocytes, zygotes and 2-cell embryos ( Fig. 4 ). Whereas Tet1 expression can barely be detected in oocytes and zygotes [14] and Tet2 is only moderately expressed, Tet3 shows extremely high levels of expression confined to oocytes and zygotes, but is nearly absent at the 2-cell stage. Hence, enzymes that are potentially responsible for the dynamic generation of 5hmC are present in the zygote/oocyte. 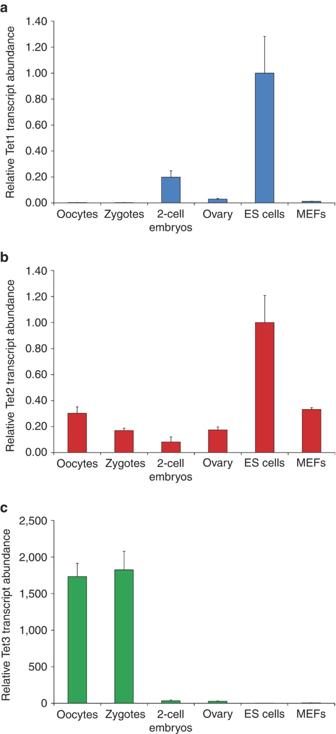Figure 4: Relative expression of Tet transcripts in development. Levels of Tet1 (a), Tet2 (b) and Tet3 (c) mRNA were measured by qRT–PCR. ES cells were used as calibrator sample (expression set to 1). The results are the average of three replicates with error bars (s.e.m.). Figure 4: Relative expression of Tet transcripts in development. Levels of Tet1 ( a ), Tet2 ( b ) and Tet3 ( c ) mRNA were measured by qRT–PCR. ES cells were used as calibrator sample (expression set to 1). The results are the average of three replicates with error bars (s.e.m.). Full size image RNA interference knockdown of Tet proteins diminishes loss of 5mC Using an RNA interference-based strategy similar to the one described by Okada et al . [19] we ablated Tet1-3 by injecting short interfering RNAs (siRNAs) against Tet mRNAs into MII oocytes followed by intracytoplasmic sperm injection fertilization ( Fig. 5a ). Scrambled siRNAs with the same base composition were used as controls. 5hmC IF staining of zygotes fixed at G2-phase after injection of siRNAs against all three Tet proteins revealed a substantial reduction of 5hmC signals in both parental pronuclei compared with the control group ( Fig. 5b–d ). Consistent with the almost exclusive expression of Tet3 in the zygote, injection of Tet3 siRNAs alone yielded similar results. We conclude that Tet3 contributes significantly to the generation of 5hmC in the mammalian zygote. Most strikingly, both Tet1–3 and Tet3 siRNA injections also affect the presence 5mC signals in the paternal pronucleus ( Fig. 5e, f ). In the paternal pronucleus, the 5mC content is strongly increased compared with control samples. This finding directly links the loss of 5mC signals to the conversion of 5mC into 5hmC. In zygotes injected with Tet3 siRNA this mechanism is disturbed. In contrast to the dramatic changes in the paternal pronucleus, the Tet knockdowns had only a mild and insignificant effect on the 5mC signal in the maternal pronucleus ( Fig. 5d ). We conclude that the vast majority of 5mC in the maternal pronucleus is inaccessible for Tet3-mediated oxidation. 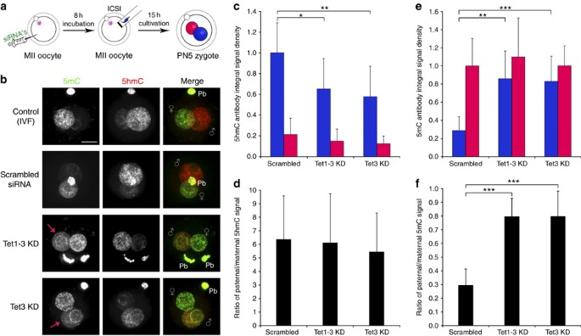Figure 5: Ablation of Tet proteins diminishes the loss of 5mC signal in the paternal genome of G2-phase zygotes. (a) Experimental setup according to Okadaet al.19. Briefly, siRNA injected metaphase II oocytes were cultured for 8 h and fertilized by intracytoplasmic sperm injection (ICSI). G2-phase zygotes were fixed and analysed for 5mC and 5hmC by immunofluorescence. (b) Representative images of 5mC (green mouse monoclonal, gift from Dirk Schübeler) and 5hmC (red rabbit polyclonal from Active Motif) immunostainings on G2-stage zygotes derived from Tet1-3 siRNA injected oocytes fertilized by ICSI. As control IVF-derived zygotes and zygotes derived from scrambled siRNA injected and ICSI fertilized oocytes are shown. Red arrows indicate the diminished loss of 5mC signal in paternal pronuclei of Tet KD-derived zygotes. Note the decreased 5hmC signal in Tet1–3 and Tet3 KDs. (c) Quantification of 5hmC signal of G2-phase zygotes derived from scrambled and Tet siRNA injected oocytes. (d) Paternal to maternal pronuclear 5hmC signal ratios. (e) Quantification of 5mC signal of G2-phase zygotes derived from scrambled and Tet siRNA injected oocytes. (f) Paternal to maternal pronuclear 5mC signal ratios. Blue bars represent signals from paternal pronuclei and red bars represent signals from maternal pronuclei. A total of 8–9 precisely staged ICSI-derived zygotes per group were analysed. Asterisks show significant changes of paternal or maternal 5hmC/5mC signals calculated using Student'st-tests (*=P<0.05, **=P<0.01, ***=P<0.001). Error bars represent standard deviations. ♂, male pronucleus; ♀, female pronucleus; Pb, polar body; scale bar, 20 μm. Figure 5: Ablation of Tet proteins diminishes the loss of 5mC signal in the paternal genome of G2-phase zygotes. ( a ) Experimental setup according to Okada et al . [19] . Briefly, siRNA injected metaphase II oocytes were cultured for 8 h and fertilized by intracytoplasmic sperm injection (ICSI). G2-phase zygotes were fixed and analysed for 5mC and 5hmC by immunofluorescence. ( b ) Representative images of 5mC (green mouse monoclonal, gift from Dirk Schübeler) and 5hmC (red rabbit polyclonal from Active Motif) immunostainings on G2-stage zygotes derived from Tet1-3 siRNA injected oocytes fertilized by ICSI. As control IVF-derived zygotes and zygotes derived from scrambled siRNA injected and ICSI fertilized oocytes are shown. Red arrows indicate the diminished loss of 5mC signal in paternal pronuclei of Tet KD-derived zygotes. Note the decreased 5hmC signal in Tet1–3 and Tet3 KDs. ( c ) Quantification of 5hmC signal of G2-phase zygotes derived from scrambled and Tet siRNA injected oocytes. ( d ) Paternal to maternal pronuclear 5hmC signal ratios. ( e ) Quantification of 5mC signal of G2-phase zygotes derived from scrambled and Tet siRNA injected oocytes. ( f ) Paternal to maternal pronuclear 5mC signal ratios. Blue bars represent signals from paternal pronuclei and red bars represent signals from maternal pronuclei. A total of 8–9 precisely staged ICSI-derived zygotes per group were analysed. Asterisks show significant changes of paternal or maternal 5hmC/5mC signals calculated using Student's t -tests (*= P <0.05, **= P <0.01, ***= P <0.001). Error bars represent standard deviations. ♂, male pronucleus; ♀, female pronucleus; Pb, polar body; scale bar, 20 μm. Full size image PGC7 protects the maternal genome against hydroxylation The maintenance of 5mC in the maternal pronucleus was shown to depend on the 'demethylation' protecting factor PGC7/Dppa3/Stella [20] . To test, whether generation of 5hmC is also influenced by PGC7, we examined the presence of 5hmC in the maternal pronucleus of mouse zygotes with a maternal null allele for PGC7 ( Fig. 6 ). Indeed, in the absence of PGC7 the maternal 5hmC signal increases substantially, whereas the 5mC signal decreases simultaneously. This finding suggests that PGC7 shields the 5mC from the Tet3-mediated oxidation. 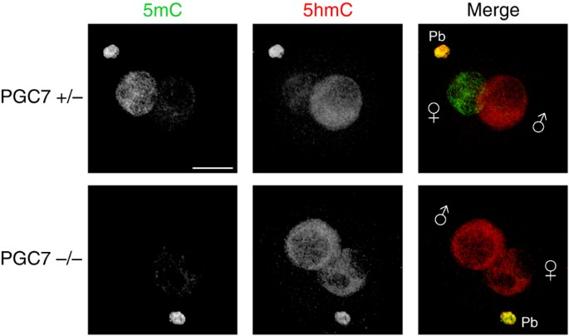Figure 6: Increase of 5hmC in the maternal genome of zygotes derived from PGC7-null oocytes. Representative images of G2-phase zygotes obtained from PGC7-null female mice stained with 5mC (green mouse monoclonal from calbiochem) and 5hmC (red rabbit polyclonal from Active Motif) antibodies (N>20). ♂, male pronucleus; ♀, female pronucleus; Pb, polar body; scale bar, 20 μm. Figure 6: Increase of 5hmC in the maternal genome of zygotes derived from PGC7-null oocytes. Representative images of G2-phase zygotes obtained from PGC7-null female mice stained with 5mC (green mouse monoclonal from calbiochem) and 5hmC (red rabbit polyclonal from Active Motif) antibodies ( N >20). ♂, male pronucleus; ♀, female pronucleus; Pb, polar body; scale bar, 20 μm. Full size image Our results reveal an important role of 5hmC in genome-wide DNA methylation reprogramming. First and most importantly, we detect 5hmC as a highly abundant modification in the paternal pronucleus of mammalian zygotes. The presence and the parental asymmetry found in the three species point towards an evolutionary conserved role of this modification in DNA methylation reprogramming. The accumulation of 5hmC during the first cell cycle does apparently not continue in the 2-cell stage and the parental asymmetry of 5hmC appears to remain across the first cleavage. This indicates that 5hmC is a rather stable modification of early cleavage stages. It remains an open and very interesting question, how 5hmC affects the maintenance and de novo DNA methylation function of DNA methyltransferases. A second major finding of our work concerns the mechanisms of 5hmC generation. Our Tet3 knockdown experiments show that 5hmC is apparently generated by a direct conversion of 5mC catalysed by this dioxygenase. Tet3 is strongly expressed in oocytes and zygotes, but this expression significantly decreases in 2-cell embryos in line with the observation that we do not observe a further increase in 5hmC levels. The Tet knockdown effects in the zygote directly link the rapid active loss/demethylation of 5mC to its conversion into 5hmC. Third, the conversion of 5mC to 5hmC by Tet3 seems to be the dominant 'default' pathway in oocytes. Nuclei of cumulus cells transferred into enucleated oocytes (SCNT embryos) show a strong increase on their 5hmC content. Hence, the Tet-mediated conversion of 5mC to 5hmC is not a specific hallmark of decondensed sperm DNA alone. The question remains, what distinguishes paternal (and somatic) chromatin from the maternal genome as substrates for Tet3-mediated 5mC conversion. Our analysis shows that PGC7 has an important role in this process. In the maternal pronucleus, the Tet3-mediated oxidation is apparently blocked/inhibited by the presence of PGC7. In the absence of PGC7, the high 5mC content of the maternal genome can be converted into 5hmC. How PGC7 exactly confers this protection remains unclear, but it seems likely that a particular chromatin composition of the maternal chromatin is required for this function. How do the findings of an extensive loss of 5mC by conversion into 5hmC reconcile with previous results and interpretations on DNA-demethylation mechanisms [7] , [21] , [22] , [23] ? Several lines of evidence suggested that base excision repair processes are associated with early pre-replicative phases of DNA demethylation. Bisulphite analyses on early zygotic stages (PN1 to early PN3), however, only revealed a moderate decrease of modified cytosines [7] (note that bisulphite sequencing does not distinguish between 5mC and 5hmC). This indicates that a small but detectable fraction of 5mC is (directly) converted into cytosine by repair-coupled processes. It is tempting to speculate that the increased levels of 5hmC may well serve as an intermediate modification recognized by active, repair coupled demethylation processes either involving a deamination or a direct DNA glycosylase-induced repair [9] . Indeed, mid to late stage paternal pronuclei, that is, pronuclei which contain extensive 5hmC and reduced 5mC levels show increased signatures of DNA strand breaks and repair markers [7] , [23] . It is also conceivable that Tet enzymes or other oxygenases may catalyse a further enzymatic oxidation of the 5hmC intermediate, leading to decarboxylation reaction and finally a demethylated unmodified cytosine. However, our data suggest that 5hmC may not only serve as an intermediate modification that triggers active DNA-demethylation. The accumulation of 5hmC in the zygote and its persistence in the 2-cell stage point towards a relative stability of this modification. The generation of 5hmC may be linked to chromatin (re)organization events in early cleavage embryos, which mainly but not exclusively occurs in the paternal genome. On the molecular level, the conversion of 5mC into 5hmC is likely to interfere with the recognition and binding of 5mC recognizing proteins [24] (MBDs, NP95, Dnmt1 and so on) and, hence, directly or indirectly influence the transcriptional rate or DNA replication associated maintenance of DNA methylation. Recent data already point towards an important regulatory role of Tet1- and Tet2-mediated oxidation for ES cell development and maintenance of pluripotency [14] , [25] , [26] . A detailed molecular profiling of 5hmC during early cleavage stages and a genetic analysis of candidate modifiers such as Tet3 will certainly elucidate the biological functions of 5hmC for early development. IVF of mouse oocytes All animal experiments were carried out according to the German Animal Welfare law in agreement with the authorizing committee. Spermatozoa collection and IVF procedures were carried out as described [27] . Briefly, sperm was isolated from the cauda epididymis of adult F1(C57BL/6×DBA) male mice and capacitated by pre-incubation for 1.5 h in pre-gassed modified KSOM medium (Millipore) supplemented with 30 mg ml −1 BSA. Mature oocytes were collected 14 h post-human chorionic gonadotropin (hCG) injection of adult F1(C57BL/6×DBA) female mice according to the standard procedures [27] . Cumulus–oocyte complexes (COCs) were placed into a 400 μl drop of KSOM medium with capacitated sperm and incubated at 37 °C in a humidified atmosphere of 5% CO 2 and 95% air. Zygotes were collected at several time points corresponding to pronuclear stages from PN0 up to metaphase stage. The classification of PN stages was done according to Adenot et al . [27] and Santos et al ., [6] in which the pronuclear morphology and hours post-fertilization are taken into consideration [6] , [28] . After brief washing in M2 medium, zona pellucida was removed by treatment with acidic tyrodes solution [27] . Subsequently, the zygotes were fixed for 20 min in 3.7% paraformaldehyde in PBS at 4 °C and permeabilized with 0.2% Triton X-100 in PBS for 10 min at room temperature (RT). The fixed zygotes were blocked overnight at 4 °C in 1% BSA, 0.1% Triton X-100 in PBS. For inhibition of DNA replication, IVF-derived zygotes were incubated with 3 μg ml −1 aphidicolin starting from 7 h.p.f. up to 14 h.p.f. IVF of bovine oocytes Bovine embryos were produced by in vitro maturation and fertilization of oocytes as previously described [29] . Briefly, cumulus–COCs were isolated from ovaries obtained from a local slaughterhouse. COCs were washed three times in culture medium TCM 199 (Seromed) supplemented with L -glutamine (100 mg l −1 ), NaHCO 3 (3 g l −1 ), HEPES (1400 mg l −1 ), sodium pyruvate (250 mg l −1 ), L -lactic-calcium salt (600 mg l −1 ) and gentamicin (55 mg l −1 ; Seromed). Oocytes were transferred to four-well plates (Nunc) with 400 ml TCM 199 supplemented with 10% oestrous cow serum and containing 0.2 U ml −1 o-FSH (Ovagen; ICPbio). Oocytes were matured for 20–22 h at 39 °C in an atmosphere of 5% CO 2 and maximum humidity. Matured COCs were washed three times in fertilization medium (Tyrode albumin lactate pyruvate) supplemented with sodium pyruvate (2.2 mg ml −1 ), heparin sodium salt (2 mg ml −1 ), and BSA (6 mg ml −1 ) and transferred to 400-ml droplets of medium. Frozen-thawed spermatozoa were subjected to the swim-up procedure for 90 min. Then the COCs and spermatozoa (2×10 6 cells per ml) were co-incubated for 18 h in maximum humidity, 39 °C and 5% CO 2 in air. The presumptive zygotes were mechanically denuded by vortexing, washed three times in synthetic oviductal fluid culture medium enriched with 10% oestrous cow serum, BME 100× (20 ml ml −1 ; Invitrogen) and MEM (minimum essential medium) 100× (10 ml ml −1 , Invitrogen) and transferred to 400-ml droplets of medium covered with mineral oil (Sigma-Aldrich). The culture atmosphere was 5% CO 2 , 5% O 2 , 90% N 2 and 39 °C at maximum humidity. In vivo rabbit embryo production Rabbit embryos were collected from superovulated outbred Zika rabbits mated with Zika males as described previously [30] . Briefly, female rabbits were superovulated by injection of 100 IU eCG (Intergonan; Intervet) intramuscularly and 100 IU hCG (Ovogest 1500; Intervet) intravenously 72 h later and mated immediately after hCG injection. For recovery of zygotes, females were killed 16 h after mating and laparotomized. The oviducts were flushed and the fertilized oocytes transferred into 100-ml drops of MPM medium supplemented with 10% (v/v) fetal calf serum (Biochrom), covered with mineral oil and cultured at 39 °C in a humidified atmosphere of 5% CO 2 , 5% O 2 and 90% N 2 (ref. 31 ). Embryos were cultured up to the G2-phase stage and fixed as described above. Embryo staining and immunofluorescence microscopy For the 5hmC and 5mC staining, fixed zygotes were incubated in 4 N HCl solution at RT for 15 min. Following neutralization (10 min 100 mM Tris-HCl, pH 8.0) and second fixation, the embryos were stained with anti-5hmC (two different antibodies, rabbit polyclonal from Active Motif (1/100) or rat monoclonal Ab 63.3 from W.R. and Adrian Bird (20 μg ml −1 ), available from Diagenode), anti-5mC (mouse monoclonal, gift from Dirk Schübeler (0.2 μg ml −1 ) and Calbiochem (1/2000)) and anti-ssDNA (mouse monoclonal from Millipore (0.5 μg ml −1 ) or rabbit polyclonal from Immuno-Biological Laboratories (0.5 μg ml −1 )). Followed by several washes in blocking solution the embryos were incubated at RT with anti-mouse or -rat secondary antibodies for 2 h coupled with Alexa Fluor 488 (10 μg ml −1 ) or 568 (10 μg ml −1 ; Molecular Probes) and anti-rabbit secondary antibodies coupled with Rhodamine Red-X (15 μg ml −1 , Jackson ImmunoResearch Laboratories). Zygotes were then washed and mounted on slides with a small drop of Vectashield (VectorLab) mounting medium. The embryos were analysed on Zeiss Axiovert 200M inverted microscope (Zeiss) as described [7] . ImageJ software was used to quantify antibody signals of z-stack computed ( ∼ 20 stacks with 0.4 μm per sample) IF images. Somatic cell nuclear transfer MII oocytes were collected from superovulated B6C3F1 mice, 14 h post-hCG administration. Oviducts were dissected in HEPES-Chatot, Ziomet, and Bavister (H-CZB) medium containing 50 IU ml −1 hyaluronidase for 20′; denuded MII oocytes were washed in α-MEM, BSA 0.2% and cultured for 30′ in α-MEM at 37 °C in 5% CO 2 . Enucleation was performed in H-CZB containing 5 μg ml −1 cytochalasin B and 0.1% polyvinylpyrrolidon (PVP). Groups of 20 oocytes were enucleated in a time window of 10′ and then extensively washed and returned to the incubator in a drop of α-MEM, 0.2% BSA. Nuclear transfer was done in 90% H-CZB, 1% PVP. Reconstructed embryos were left to recover for at least 1 h in α-MEM in the incubator before being chemically activated in Ca 2+ -free α-MEM, SrCl 2 10 mM in the presence of 5 μg ml −1 cytochalasin B and 0.05% DMSO [32] . At different time points embryos were collected and fixed for further immunostaining. Analysis of zygotes derived from PGC7−/− oocytes PGC7+/− and PGC7−/− female mice >8-weeks old were superovulated by injecting 5 U of hCG 48 h after a 5 U injection of pregnant mare serum gonadotropin and then mated with stud male mice. Zygotes were collected from the oviduct after 28 h hCG injection and were analysed by immunostaining as described. The zygotes were mounted on slides with Mountant Permafluor (Lab Vision). IF was visualized using an LSM510 confocal laser scanning microscope (Carl Zeiss). Expression analysis of Tet RNAs Total RNA was isolated from mouse oocytes ( n =20, B6×SD7), zygotes ( n =74, B6×SD7), two-cell embryos ( n =33), ovary, ES cells (E14) and primary mouse embryonic fibroblasts (passage 3) using Trizol reagent (Invitrogen) supplemented with 60 μg of mussel glycogen (Roche) for oocyte/embryo samples. cDNA was analysed by qRT–PCR using standard conditions. Ct values used for calculating relative expression were the average of three replicates and were normalized against two reference genes ( Atp5b and Hsp90ab1 ). The primers used are as follows: Atp5b F—5′-ggccaagatgtcctgctgtt-3′; Atp5b R—5′-gctggtagcctacagcagaagg-3′; Hsp F—5′-gctggctgaggacaaggaga-3′; Hsp R—5′-cgtcggttagtggaatcttcatg-3′; Tet1 F—5′-ccattctcacaaggacattcaca-3′; Tet1 R—5′-gcaggacgtggagttgttca-3′; Tet2 F—5′-gccattctcaggagtcactgc-3′; Tet2 R—5′-acttctcgattgtcttctctattgagg-3′; Tet3 F—5′-ggtcacagcctgcatggact-3′; Tet3 R—5′-agcgattgtcttccttggtcag-3′. Annealing temperatures of 58 °C were used for all primer sets. Dissociation curves were performed to confirm specificity of the PCR products and relative expression was calculated with qBase software [33] . Tet knockdown experiments Experimental setup was done according to Okada et al . [19] siRNAs (2 μM each) were co-injected with Dextran-tetramethyl-rhodamine (Invitrogen, 3000 MW, 100 μg ml −1 ) in MII arrested oocytes derived from superovulated F1(C57BL/6×DBA) mice. After 8 h of incubation at 37 °C in a humidified atmosphere of 5% CO2 and 95% air, siRNA injected oocytes were fertilized by intracytoplasmic sperm injection. After 15 h of cultivation, G2-phase zygotes were fixed and analysed for 5mC and 5hmC by immunostaining as described. Quantification of 5mC and 5hmC signals was done as described. siRNA target sequences are listed in Supplementary Table S1 . How to cite this article : Wossidlo, M. et al . 5-Hydroxymethylcytosine in the mammalian zygote is linked with epigenetic reprogramming. Nat. Commun. 2:241 doi: 10.1038/ncomms1240 (2011).